Topological quantum computing with a very noisy network and local error rates approaching one percent A scalable quantum computer could be built by networking together many simple processor cells, thus avoiding the need to create a single complex structure. The difficulty is that realistic quantum links are very error prone. A solution is for cells to repeatedly communicate with each other and so purify any imperfections; however prior studies suggest that the cells themselves must then have prohibitively low internal error rates. Here we describe a method by which even error-prone cells can perform purification: groups of cells generate shared resource states, which then enable stabilization of topologically encoded data. Given a realistically noisy network (≥10% error rate) we find that our protocol can succeed provided that intra-cell error rates for initialisation, state manipulation and measurement are below 0.82%. This level of fidelity is already achievable in several laboratory systems. Topological codes are an elegant and practical method for representing information in a quantum computer. The units of information, or logical qubits, are encoded as collective states in an array of physical qubits [1] . By measuring stabilizers, that is, properties of nearby groups of physical qubits, we can detect errors as they arise. Moreover, with a suitable choice of stabilizer measurements we can even manipulate the encoded qubits to perform logical operations. The act of measuring stabilizers over the array thus constitutes a kind of ‘pulse’ for the computer—it is a fundamental repeating cycle and all higher functions are built upon it. In the idealised case that the stabilizer measurements are performed perfectly, we can recover the logical qubit from a very corrupt topological memory (for example in the toric code ∼ 19% of the physical qubits can be corrupt [2] ). However, in a real device the stabilizer measurements will sometimes introduce errors, due to failures while initialising ancillas, performing gate operations or measurements. Will the act of measuring stabilizers still ‘do more good than harm’ and protect the encoded information? This depends on the frequency of such errors; estimates of the threshold error rate are 0.75–1.4% depending on the model [3] , [4] , [5] . These numbers are applicable to a ‘monolithic’ architecture, but for many systems a network architecture may be more scalable ( Fig. 1 ). Links will be error prone, but cells can interact repeatedly and purify the results to remove errors [6] , [7] . Thus one can realise a ‘noisy network’ (NN) paradigm, also called distributed [8] , [9] or modular [10] . However prior analyses of this approach have indicated a serious drawback. The need to perform purification means a cell’s own internal error rate must be very low; of the 0.1% order [6] , [7] , [8] , [9] , [10] . Given that a real machine should operate well below threshold, such a demand may be prohibitive. It is timely to seek a less demanding approach, given that entanglement over a remote link has now been demonstrated with NV centres [11] , adding diversity to the previous atomic experiments [12] . 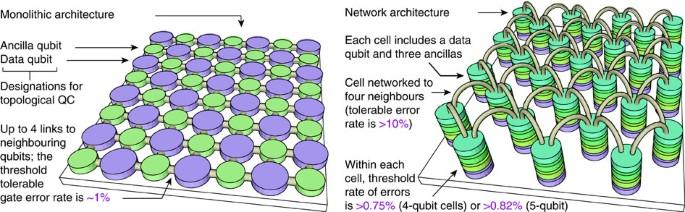Figure 1: Quantum architectures. Left: a monolithic grid of qubits with neighbours directly connected to enable high fidelity two-qubit operations. (layout from ref.5.) Such a structure is a plausible goal for some systems, for example, specific superconducting devices23. Right: For other nascent quantum technologies the network paradigm is appropriate. A single nitrogen-vacancy (NV) centre in diamond, with its electron spin and associated nuclear spin(s)24, would constitute a cell. A small ion trap holding a modest number of ions10,25is another example. Noisy network links with error rates ≥ 10% are acceptable. For photonic links this goal is realistic given imperfections like photon loss and instabilities in path lengths or interaction strengths. Similarly, with solid state ‘wires’ formed by spin chains26, noisy entanglement distribution of this kind is a reasonable goal27. Figure 1: Quantum architectures. Left: a monolithic grid of qubits with neighbours directly connected to enable high fidelity two-qubit operations. (layout from ref. 5 .) Such a structure is a plausible goal for some systems, for example, specific superconducting devices [23] . Right: For other nascent quantum technologies the network paradigm is appropriate. A single nitrogen-vacancy (NV) centre in diamond, with its electron spin and associated nuclear spin(s) [24] , would constitute a cell. A small ion trap holding a modest number of ions [10] , [25] is another example. Noisy network links with error rates ≥ 10% are acceptable. For photonic links this goal is realistic given imperfections like photon loss and instabilities in path lengths or interaction strengths. Similarly, with solid state ‘wires’ formed by spin chains [26] , noisy entanglement distribution of this kind is a reasonable goal [27] . Full size image Here we describe a new NN protocol which achieves a threshold for the intra-cell operations which is far higher, and comparable to current estimates for tolerable noise in monolithic architectures. Our cells collectively represent logical qubits according to the 2D toric code (one of the simplest and most robust topological surface codes). This code is stabilized by repeatedly measuring the parity of groups of four qubits in either the Z or the X basis. In our approach each elementary ‘data qubit’ of the code resides in a separate cell, alongside a few dedicated ancilla qubits. We implement stabilizer measurements by directly generating a GHZ state shared across the ancillas in four cells, before consuming this resource in a single step to measure the stabilizer on the four data qubits. This procedure is in the spirit of the bandaid protocol [13] and contrasts with the standard approach of performing a sequence of two-qubit gates between the four data qubits and a fifth auxiliary qubit (which, in the network picture, would require its own cell). By directly generating the GHZ state over the network we remove the need for the auxiliary unit and more importantly we can considerably reduce the accumulation of errors. Protocol In this paper we consider three variants of our noisy network protocol. In all cases, one qubit in each cell is designated the data qubit and the others are ancillas that will be initialised, processed and measured during each stabilizer evaluation process. 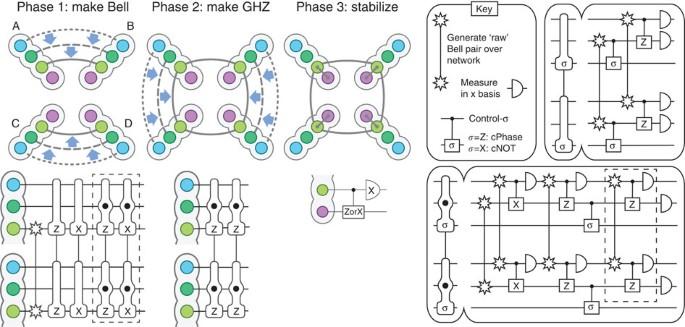Figure 2: Protocols for stabilizer measurement. The three phases for generating and consuming a 4-cell GHZ state among the ancilla qubits (blue-to-green) in order to perform a stabilizer measurement on the data qubits (purple). Phase (1): use purification to create a high quality Bell pair shared between cell A and cell B, while in parallel doing the same thing with cells C and D. (2) Fusion operations, A to C and B to D, create a high fidelity GHZ state. (3) Finally use the GHZ state to perform a one-step stabilizer operation. The parity of the four measured classical bits is also the parity of the stabilizer operation we have performed on the data qubits. Two dashed regions indicate operations that are part of the STRINGENT protocol; omitting them yields the EXPEDIENT alternative. Figure 2 defines two of the variants: if we neglect the elements enclosed in dashed lines then we have the compact EXPEDIENT protocol, meanwhile applying all steps yields the STRINGENT alternative. The former has the advantage that it requires less time to perform. Presently we also introduce a further protocol called STRINGENT+ which requires an additional qubit in each cell. Establishing the performance of these three variants is the principle aim of this paper. The results are detailed presently; in summary, setting the network error rate to 10% one finds threshold local error rates of about 0.6, 0.775 and 0.825% for EXPEDIENT, STRINGENT and STRINGENT+ respectively. Optionally we can trade local error rate for still greater network noise tolerance, see Supplementary Note 1 . These thresholds are considerably higher than those in prior work; for example in a recent paper [8] we applied an optimised purification protocol [14] to the case of a network with three qubits per node, finding a threshold local error rate in the region of 0.1%. The improved rates seen in the present paper result from generating and purifying a GHZ resource state over the network, followed by a one-step stabilizer measurement. It seems that the additional storage in this new method requires at least four qubits per cell. Figure 2: Protocols for stabilizer measurement. The three phases for generating and consuming a 4-cell GHZ state among the ancilla qubits (blue-to-green) in order to perform a stabilizer measurement on the data qubits (purple). Phase (1): use purification to create a high quality Bell pair shared between cell A and cell B, while in parallel doing the same thing with cells C and D. (2) Fusion operations, A to C and B to D, create a high fidelity GHZ state. (3) Finally use the GHZ state to perform a one-step stabilizer operation. The parity of the four measured classical bits is also the parity of the stabilizer operation we have performed on the data qubits. Two dashed regions indicate operations that are part of the STRINGENT protocol; omitting them yields the EXPEDIENT alternative. Full size image We assume the network channel between two cells can create shared, noisy Bell pairs in the Werner form where . Throughout this paper unless otherwise stated we take the network error probability to be p n =0.1. This ‘raw’ Bell generation is the sole operation that occurs over the network. We additionally require only three intra-cell operations: controlled- Z (that is, the two-qubit phase gate), controlled- X (that is, the control-NOT gate) and single qubit measurement in the X -basis. The two qubit gates are modelled in the standard way: an ideal operation followed by the trace-preserving noise process where operator acts on the first qubit, and similarly B acts on the second qubit, but we exclude the case ⊗ from the sum. Meanwhile noisy measurement is modelled by perfect measurement preceded by inversion of the state with the probability p m . Phases 1 and 2 in Fig. 2 are postselective: whenever we measure a qubit, one outcome indicates ‘continue’ and the other indicates that we must recreate the corresponding resource (the desired outcome is that which we would obtain, were the noise parameters set to zero). We note that in the circuits developed here we adopt and extend the ‘double selection’ concept introduced by Fujii and Yamamoto in ref. 15 . Resource overhead can be quite modest: EXPEDIENT minimises the number of raw pairs required and thus the overall time requirement. On average it requires fewer than twice the number of pairs consumed in the ideal case that all measurements ‘succeed’, see Supplementary Note 2 . Performance evaluation Having specified the stabilizer measurement protocols, we must determine their real effect given the various error rates p n , p g and p m . It is convenient derive a single superoperator describing the action of the entire stabilizer protocol on the four data qubits. This is described in the Methods section below. Given this operator, together with a suitable scheduling scheme as shown in Fig. 3 , we proceed to determine thresholds by intensive numerical modelling. Our model introduces errors randomly but with precisely the correct correlation rates. We record the (noisy) stabilizer outcomes and subsequently employ Edmonds’ minimum weight perfect matching algorithm [16] , implemented as described in ref. 17 , to pair and resolve stabilizer flips in the standard way (see for example, ref. 5 ). This technique allows us to establish the threshold for successful protection of quantum information by simulating networks of various sizes. If an increase of the network size allows us to protect a unit of quantum information more successfully, then we are below threshold. Conversely if increasing the network size makes things worse, then in effect the stabilizers are introducing more noise than they remove and we are above threshold. The results of a large number of such simulations are shown in Fig. 4 (and equivalent data for the monolithic case are shown in Supplementary Fig. S1 ). In these Figures we sweep the local error rate to determine the threshold; equivalently one can sweep the network error rate as shown in Supplementary Fig. S2 . We see thresholds for EXPEDIENT and for STRINGENT of over 0.6 and 0.77% respectively. The third graph shows the performance of a five-qubit-per-cell variation of STRINGENT which we describe in more detail in the Supplementary Note 1 . It achieves a threshold in excess of 0.82% by employing an additional filter such that most stabilizer measurements are improved while a known minority become more noisy, and this classical information is fed into an enhanced Edmonds’ algorithm. 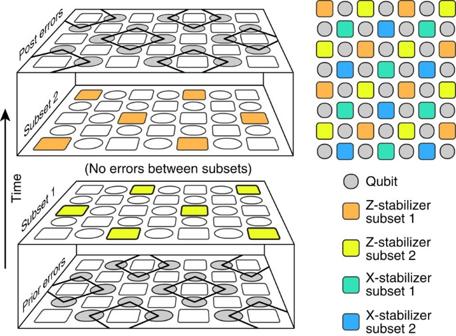Figure 3: Scheduling stabilizer operations. The right side graphic shows the standard arrangement of one complete stabilizer cycle, involvingZandXprojectors (square symbols indicate that the four surrounding data qubits are to be stabilized). Because a given cell can only be involved in generating one GHZ resource at a given time, each of these two stabilizer types must be broken into two subsets; see main figure. Fortunately in our stabilizer superoperator we can commute projectors and errors so as to expel errors from the intervening time between subsets, so allowing them to merge. Figure 3: Scheduling stabilizer operations. The right side graphic shows the standard arrangement of one complete stabilizer cycle, involving Z and X projectors (square symbols indicate that the four surrounding data qubits are to be stabilized). Because a given cell can only be involved in generating one GHZ resource at a given time, each of these two stabilizer types must be broken into two subsets; see main figure. Fortunately in our stabilizer superoperator we can commute projectors and errors so as to expel errors from the intervening time between subsets, so allowing them to merge. 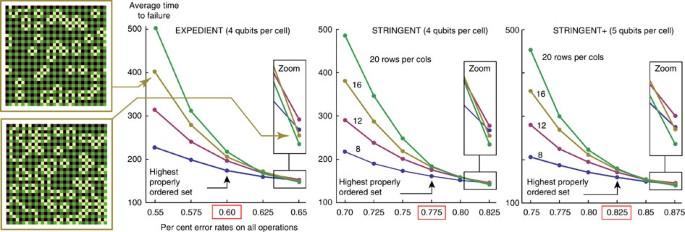Figure 4: Performance of the EXPEDIENT and STRINGENT protocols. We employ a toric code withnrows ×ncolumns of data qubits (2n2in total). A given numerical experiment is a simulation of 100 complete stabilizer measurement cycles on an initially perfect array, after which we attempt to decode aZmeasurement of the stored qubit. The result is either a success or a failure; for each data point we perform at least 10,000 experiments to determine the fail probability, and reciprocate this to infer an expected time to failure. Network error rates are 10% in all cases; we set intra-cell gate and measurement error rates equal,pm=pg, and plot this on the horizontal axes. For low error rates the system’s performance improves with increasing array size. As the error rates pass the threshold this property fails. Insets: typical final states of the toroidal array after error correction. Yellow squares are flipped qubits, green squares indicate the pattern of Z-stabilizers. Closed loops are successful error corrections; while both arrays are therefore successfully corrected, it is visually apparent that the above-threshold case is liable to long paths. Full size image Figure 4: Performance of the EXPEDIENT and STRINGENT protocols. We employ a toric code with n rows × n columns of data qubits (2 n 2 in total). A given numerical experiment is a simulation of 100 complete stabilizer measurement cycles on an initially perfect array, after which we attempt to decode a Z measurement of the stored qubit. The result is either a success or a failure; for each data point we perform at least 10,000 experiments to determine the fail probability, and reciprocate this to infer an expected time to failure. Network error rates are 10% in all cases; we set intra-cell gate and measurement error rates equal, p m = p g , and plot this on the horizontal axes. For low error rates the system’s performance improves with increasing array size. As the error rates pass the threshold this property fails. Insets: typical final states of the toroidal array after error correction. Yellow squares are flipped qubits, green squares indicate the pattern of Z-stabilizers. Closed loops are successful error corrections; while both arrays are therefore successfully corrected, it is visually apparent that the above-threshold case is liable to long paths. Full size image External decoherence We have yet to consider general decoherence caused by the external environment during a stabilizer protocol. Fortunately many of the systems most relevant to the NN approach have excellent low-noise ‘memory qubits’ available. For example in NV centres at room temperature, nuclear spins can retain coherence for the order of a second; and for impurities in silicon the record is several minutes [18] , [19] . We would naturally use such spins for our data qubits and for the innermost ancilla qubits, that is, those bearing the GHZ-state in Fig. 2 . In Supplementary Note 3 we summarise the relevant control and measurement timescales from recent NV centre and atomic experiments, and thus estimate the probability of an environmentally induced error during a full stabilizer protocol. We find that such error probabilities are small compared to the error rates p g and p m that we have already considered. Computation versus qubit storage The results described here are thresholds for successful protection of encoded logical qubits. We do not explicitly simulate the act of performing a computation involving two or more logical qubits. However it is generally accepted that the threshold for full computation will be very similar to that for successful information storage, because the stabilizer measurements required for simple preservation of the encoded state are very similar to those required for computation [3] , [20] . In both cases, the standard four-qubit stabilizer is overwhelmingly the most common measurement. For computation it is necessary to evaluate additional forms of stabilizer, for example a stabilizer measurement corresponding to the ( X or Z -basis) parity of three, rather than four, qubits. This applies both in the approach of braiding defects [3] and the alternative idea of performing ‘lattice surgery’ [20] . However these alternative stabilizers are a minority, being required at boundaries while the four-qubit standard stabilizer still forms the bulk of operations. Moreover both for monolithic architectures and the noisy network paradigm, the three-qubit stabilizer will in fact have a somewhat lower error rate since it requires a less complex protocol. We have described an approach to ‘noisy network’ quantum computing, where many simple modules or cells are connected with error prone links. We show that relatively high rates of error within each cell can be tolerated, while the links between the cells can be very error prone (10% or more). This work therefore largely closes the gap between error tolerance in networks versus monolithic architectures. We hope this result will encourage the several emerging technologies for which networks are the natural route to scalability; these include ion traps and NV centres (linked either optically or via spin chains). Throughout this study we have assumed that all forms of error are equally likely; in reality, in a given physical system some errors may be more prevalent. For example phase errors on the network channel might be more common than flip errors, and similarly the local gates within cells may suffer specific kinds of noise. Any such bias in error occurrences is ‘good news’ in that it can potentially be exploited by adapting our protocols, and in this way the error thresholds might be further increased. Derivation of superoperator In the following we write M to stand for the ‘odd’ or ‘even’ reported outcome of the stabilizer protocol (that is, the parity of the four measured qubits in Phase 3 of Fig. 2 ). If density matrix ρ represents the state of all data qubits prior to the evaluation of our stabilizer, then measurement outcome M and the corresponding state S M (ρ) = P M (ρ) /Tr[ P M ( ρ )] will occur with probability Tr[ P M ( ρ )], for some projective operator P M ( · ). Now stabilizing the toric code involves two types of operation, measuring the X and the Z —stabilizers. Suppose we are performing a Z stabilizer. If our protocol could act perfectly, then for example the even projector would be , where the sum is over all states | i 〉, | j 〉 with definite even parity in the Z -basis: |0000〉, |0011〉, etc. Analogously the ideal odd Z -stabilizer sums over states of definite odd parity, and meanwhile for X stabilizers the ideal projectors refer to states of definite parity in the X -basis. In reality our imperfect operations result in projectors of the form Here the four operators making up E are understood to act on data qubits 1 to 4 respectively, and index e runs over all their combinations. The symbol represents the compliment of M , that is, ‘odd’ for M =‘even’ and vice versa. We see that this real projector is made up of a mix of the correct and incorrect projectors together with possible Pauli errors; the various weights a and b capture their relative significance. Given the underlying error rates p n , p g and p m we can employ the Choi-Jamiolkowski isomorphism to find the corresponding weights { a , b } in our superoperator. Incorporated in this process is a ‘twirling’ operation; this is explained in the Supplementary Methods along with examples of the resulting weights. The largest contributor to is found to be the reported parity projection, that is, for M =‘even’, the largest of all weights { a , b } is that associated with E = and . The next largest term will be the pure ‘wrong’ projection, i.e. the combination of E = and . This form of error is relatively easy for the toric code to handle, and we have deliberately favoured it over other error types by minimising the σ x and σ y errors, rather than σ z , in our stabilizer measurement protocols. The remaining terms correspond to Pauli errors in combination with either the correct or the incorrect projectors; for example is an erroneous flip on data qubit 1 simultaneous with a phase error on qubit 2. Decoding algorithm Edmonds’ algorithm was selected, having been well studied in the context of noisy stabilizer measurements; in Supplementary Fig. S2 we apply our same model to monolithic architecture, obtaining a threshold in the region of 0.9%, generally consistent with prior studies [5] . For the idealised case of perfect (noiseless) stabilizer measurements other algorithms have been developed which may eventually offer advantages for noisy stabilizers as well [2] , [21] , [22] . How to cite this article: Nickerson, N.H. et al . Topological quantum computing with a very noisy network and local error rates approaching one percent. Nat. Commun. 4:1756 doi: 10.1038/ncomms2773 (2013).